Non-invasivein vivoassessment ofIDH1mutational status in glioma Gain-of-function mutations of the isocitrate dehydrogenase 1 ( IDH1 ) gene are among the most prevalent in low-grade gliomas and secondary glioblastoma. They lead to intracellular accumulation of the oncometabolite 2-hydroxyglutarate, represent an early pathogenic event and are considered a therapeutic target. Here we show, in this proof-of-concept study, that [1- 13 C] α-ketoglutarate can serve as a metabolic imaging agent for non-invasive, real-time, in vivo monitoring of mutant IDH1 activity, and can inform on IDH1 status. Using 13 C magnetic resonance spectroscopy in combination with dissolution dynamic nuclear polarization, the metabolic fate of hyperpolarized [1- 13 C] α-ketoglutarate is studied in isogenic glioblastoma cells that differ only in their IDH1 status. In lysates and tumours that express wild-type IDH1, only hyperpolarized [1- 13 C] α-ketoglutarate can be detected. In contrast, in cells that express mutant IDH1, hyperpolarized [1- 13 C] 2-hydroxyglutarate is also observed, both in cell lysates and in vivo in orthotopic tumours. Genetic screening has determined that over 70% of low-grade diffuse glioma tumours and up to 90% of secondary glioblastoma (GBM) cases harbour a missense point mutation in one copy of the gene encoding for the cytosolic isocitrate dehydrogenase 1 (IDH1) enzyme, most commonly at residue 132 (refs 1 , 2 ). Mutations in an equivalent residue of the mitochondrial isoform isocitrate dehydrogenase 2 have also been reported in about 20% of acute lymphoblastic leukaemia [3] . More recently, similar mutations have been observed in other cancers, including thyroid carcinomas (16%), cartilaginous tumours (75%) and intrahepatic cholangiocarcinomas (10–23%) [4] . The role and significance of mutant and wild-type IDH1 in cancer have been studied by several groups (see recent reviews in refs 5 , 6 ). Reports from clinical samples demonstrate that IDH1 mutations are monoallelic, with one copy of the wild-type gene and one copy of the mutant gene expressed in human tumours [7] . Whereas wild-type IDH1 catalyses the oxidation of isocitrate to alpha-ketoglutarate (α-KG, 2-oxoglutarate), the mutant IDH1 isoform reduces α-KG to 2-hydroxyglutarate (2-HG), resulting in 2-HG levels that are 10–100 times greater than that in wild-type tissue [1] , [2] . The interaction between wild-type and mutant enzymes is still under investigation [8] , [9] ; however, it is well established that the presence of mutant IDH1 and elevated 2-HG leads to inhibition of α-KG-dependent dioxygenases, including histone demethylases and the TET family of 5-methylcytosine hydroxylases. This, in turn, leads to genome-wide changes in histone and DNA methylation [10] , [11] . The IDH1 mutation is thus an early oncogenic event that mediates tumour development through reorganization of the methylome and transcriptome [12] , [13] . In light of its critical role in tumour pathogenesis, drugs that target mutant IDH1 are now under development [14] , [15] . In this context, non-invasive methods for real-time monitoring of IDH1 activity and modulation of 2-HG production would be valuable for tumour characterization, patient stratification and prognosis, as well as optimization of mutant IDH1 inhibitors, and subsequent longitudinal monitoring of IDH1-targeted treatments. 1 H magnetic resonance spectroscopy (MRS) is a non-invasive imaging method that can probe steady-state metabolite levels. It has been used as a diagnostic and prognostic tool in brain tumour patients [16] , [17] and is able to detect the presence of 2-HG in glioma patients in vivo [18] , [19] , [20] , [21] , in preclinical rodent models [22] , [23] and in biopsy samples [24] , [25] . An alternative, and potentially complementary, metabolic neuroimaging approach is 13 C MRS. This technique informs on real-time metabolic fluxes by probing the fate of exogenous 13 C-labelled substrates. The recent development of dissolution dynamic nuclear polarization (DNP) has allowed 13 C-labelled compounds to be hyperpolarized, dissolved into solution and injected into the sample of interest to provide a 10,000- to 50,000-fold increase in signal-to-noise ratio (SNR) compared with thermally polarized compounds [26] . 13 C MRS of hyperpolarized compounds can thus be applied to monitor in vivo enzymatic activities [27] . The conversion of hyperpolarized [1- 13 C] pyruvate to [1- 13 C] lactate has been used to detect the presence of tumour and response to treatment in several preclinical models of cancer [27] , [28] , including glioma [29] , [30] , [31] , [32] . These promising findings led to the first phase I clinical trial of this technology, which was recently completed at the University of California, San Francisco [27] , [33] . It clearly demonstrated the translational value of this approach by detecting elevated ratios of hyperpolarized lactate-to-pyruvate in tumours of prostate cancer patients. In addition to pyruvate, a number of other hyperpolarized probes have been developed to monitor other metabolic pathways, measure pH, evaluate necrosis, assess redox potential and measure vascular flow [27] . In this report, we demonstrate the successful use of a new DNP probe, [1- 13 C] α-KG, for non-invasive 13 C MRS imaging of IDH1 status. We show that, following exposure to hyperpolarized [1- 13 C] α-KG, we can detect the production of hyperpolarized [1- 13 C] 2-HG in lysates and orthotopic tumours of cells engineered to express mutant IDH1 but not in lysates or tumours of their isogenic counterparts engineered to express wild-type IDH1, nor in normal contralateral brain. We conclude that [1- 13 C] α-KG is a promising agent for the in vivo interrogation of IDH1 mutational status and activity. Characterization of hyperpolarized α-ketoglutarate To test the hypothesis that hyperpolarized [1- 13 C] α-KG can serve as an imaging probe to monitor mutant IDH1 activity ( Fig. 1a ), we first determined its achievable polarization level and its T 1 relaxation time. [1- 13 C] α-KG was mixed with a stable free radical in a 3:1 mixture of water and glycerol. After 1 h, a polarization level of 16±3% was achieved in solution at 37 °C (time constant τ =1,381 s). Following dissolution to an isotonic solution (pH=7.5±0.1, n =6), the resonances of hyperpolarized [1- 13 C] α-KG ( δ C1-αKG =172.6 p.p.m. ), [1- 13 C] α-KG hydrate ( δ αKG-H =180.9 p.p.m.) and [5- 13 C] α-KG ( δ C5-αKG =184 p.p.m., originating from the 1.1% natural abundance 13 C at the C5 position) were detected ( Fig. 1b ). 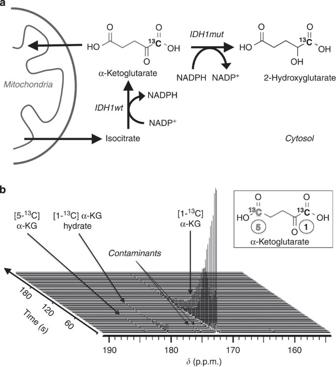Figure 1: [1-13C] α-KG is a biologically relevant DNP probe. (a) Schematic of reactions catalyzed by wild-type IDH1 (IDH1wt) and mutant IDH1 (IDH1mut), and associated [1-13C] α-KG metabolism. The13C label at the C1 position of α-KG is highlighted in bold. (b) Stack plot of13C MR spectra of hyperpolarized [1-13C] α-KG in solution acquired at 11.7 Tesla and showing decay of the hyperpolarized signals (temporal resolution 3 s, polarization level 17%). Hyperpolarized [1-13C] α-KG (δC1-αKG=172.6 p.p.m., inset black), hyperpolarized [1-13C] α-KG hydrate (δαKG-H=180.9 p.p.m.) and hyperpolarized [5-13C] α-KG (δC5-αKG=184 p.p.m., inset grey) are detectable. The in vitro T 1 values of all three resonances were determined at 3 and 11.7 Tesla ( Table 1 ). The in vitro T 1 values of hyperpolarized [1- 13 C] 2-HG were determined separately ( Table 1 ). Importantly, the lifetime of hyperpolarized [1- 13 C] α-KG at 3 Tesla was sufficiently long ( T 1 =52±4 s) that we expected to be able to probe α-KG metabolism at this field strength. Figure 1: [1- 13 C] α-KG is a biologically relevant DNP probe. ( a ) Schematic of reactions catalyzed by wild-type IDH1 (IDH1wt) and mutant IDH1 (IDH1mut), and associated [1- 13 C] α-KG metabolism. The 13 C label at the C1 position of α-KG is highlighted in bold. ( b ) Stack plot of 13 C MR spectra of hyperpolarized [1- 13 C] α-KG in solution acquired at 11.7 Tesla and showing decay of the hyperpolarized signals (temporal resolution 3 s, polarization level 17%). Hyperpolarized [1- 13 C] α-KG ( δ C1-αKG =172.6 p.p.m., inset black), hyperpolarized [1- 13 C] α-KG hydrate ( δ αKG-H =180.9 p.p.m.) and hyperpolarized [5- 13 C] α-KG ( δ C5-αKG =184 p.p.m., inset grey) are detectable. Full size image Table 1 T 1 relaxation times of 13 C-labelled compounds of interest. Full size table Studies in cell lysates U87 GBM cells were transduced with a lentiviral vector coding, respectively, for wild-type IDH1 (U87IDHwt cells), or for mutant and wild-type IDH1 (U87IDHmut cells; recapitulating the monoallelic expression observed in patient samples [7] ). Western blot analysis confirmed elevated mutant IDH1 protein in U87IDHmut cells, and elevated wild-type IDH1 in both cell lines ( Fig. 2a and Supplementary Fig. S1 ). A spectrophotometric assay confirmed the functionality of the expressed mutant IDH1 ( Fig. 2b ); the rate of NADPH consumption was almost six times higher in U87IDHmut than that in U87IDHwt cells: R U87IDHmu t =0.64±0.06 versus R U87IDHwt =0.13±0.06 fmol NADPH consumed per minute per cell (unpaired Student's t -test: P <0.01). Finally, one-dimensional (1D) 1 H MRS ( Fig. 2c ) confirmed the presence of 2-HG in U87IDHmut cell lysates, with two-dimensional (2D) 1 H MRS of the same lysates confirming the 2-HG assignment ( Fig. 2d ). The level of 2-HG U87IDHmut cells was 5.3±1.3 fmol cell −1 or 10.1±2.5 μmol g −1 assuming a cell diameter of ~10 μm. 2-HG resonances were below detection level in wild-type cells. 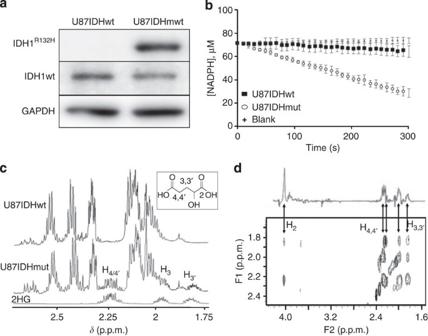Figure 2: Mutant IDH1 cells exhibit elevated enzyme activity and 2-HG levels. (a) Western blotting for wild-type IDH1 (IDH1wt, 46 kDa) and mutant IDH1 (IDH1R132H, 46 kDa) isoforms in U87IDHmut and U87IDHwt cells (GAPDH (40.2 kDa) was used as a loading control; seeSupplementary Fig. S1for full blots). (b) Spectrophotometric assay of mutant IDH1 activity in U87IDHwt (filled squares) and U87IDHmut (open circles) cells, monitoring changes in NADPH absorption over time at 340 nm compared with buffer blank (plus sign) (error bars:±s.d.m.). (c)1H spectra of pure 2-HG (bottom), U87IDHwt cell lysate (top) and U87IDHmut cell lysate (middle). Inset shows the structure of 2-HG and annotated protons detected in the spectrum. (d) Zoomed view of 2D1H total correlation spectroscopy of a U87IDHmut cell lysate acquired at 14 Tesla, illustrating the cross peaks characteristic of 2-HG (H2=4.00 p.p.m.; H3,3′=1.85/2.00 p.p.m.; H4,4′=2.25 p.p.m.). A projection representing the sum of all slices containing the 2-HG spin system is shown on top of the total correlation spectroscopy box. Figure 2: Mutant IDH1 cells exhibit elevated enzyme activity and 2-HG levels. ( a ) Western blotting for wild-type IDH1 (IDH1wt, 46 kDa) and mutant IDH1 (IDH1 R132H , 46 kDa) isoforms in U87IDHmut and U87IDHwt cells (GAPDH (40.2 kDa) was used as a loading control; see Supplementary Fig. S1 for full blots). ( b ) Spectrophotometric assay of mutant IDH1 activity in U87IDHwt (filled squares) and U87IDHmut (open circles) cells, monitoring changes in NADPH absorption over time at 340 nm compared with buffer blank (plus sign) (error bars:±s.d.m.). ( c ) 1 H spectra of pure 2-HG (bottom), U87IDHwt cell lysate (top) and U87IDHmut cell lysate (middle). Inset shows the structure of 2-HG and annotated protons detected in the spectrum. ( d ) Zoomed view of 2D 1 H total correlation spectroscopy of a U87IDHmut cell lysate acquired at 14 Tesla, illustrating the cross peaks characteristic of 2-HG (H 2 =4.00 p.p.m. ; H 3,3′ =1.85/2.00 p.p.m. ; H 4,4′ =2.25 p.p.m.). A projection representing the sum of all slices containing the 2-HG spin system is shown on top of the total correlation spectroscopy box. Full size image To show that the conversion of α-KG to 2-HG can be detected within the hyperpolarization lifetime, we first probed the fate of hyperpolarized [1- 13 C] α-KG in cell lysates. Following injection, a new resonance was detected at 183.9 p.p.m. in U87IDHmut but not in U87IDHwt cell extracts ( Fig. 3a ). This resonance was assigned to [1- 13 C] 2-HG and the assignment was further confirmed by 2D 1 H– 13 C MRS ( Fig. 3b ). Normalization to the [5- 13 C] α-KG peak (the T 1 of which is comparable, see Table 1 ) indicated that 2-HG was accumulating over time ( Fig. 3c ; the resonance of [5- 13 C] α-KG decreases not only because of T 1 relaxation but also because of conversion of α-KG to 2-HG leading to an ~2% overestimate of 2-HG production). 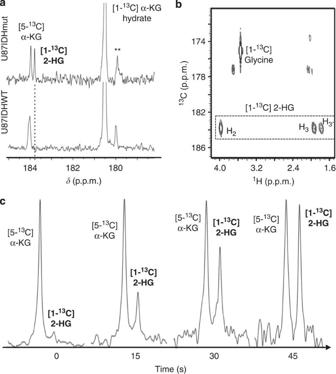Figure 3: Hyperpolarized 2-HG production is detected in mutant IDH1 cell lysates. (a)13C MR spectra acquired 45 s after injection of hyperpolarized [1-13C] α-KG in U87IDHmut cell lysate (top) and U87IDHwt cell lysate (bottom; absolute intensities; ** contaminant originating from the α-KG preparation). (b) Gradient-selected heteronuclear multiple bond coherence spectra of the same U87IDHmut lysates acquired at 14 Tesla, confirming the production of [1-13C] 2-HG from [1-13C] α-KG. The1H–13C cross peaks of [1-13C] 2-HG (dotted box), confirm the [1-13C] 2-HG assignment at 183.9 p.p.m. Note: [1-13C] glycine was used as an external reference. (c) Temporal evolution of [1-13C] 2-HG in U87IDHmut cell lysate normalized to [5-13C] α-KG peak intensity, showing build-up of hyperpolarized [1-13C] 2-HG. Figure 3: Hyperpolarized 2-HG production is detected in mutant IDH1 cell lysates. ( a ) 13 C MR spectra acquired 45 s after injection of hyperpolarized [1- 13 C] α-KG in U87IDHmut cell lysate (top) and U87IDHwt cell lysate (bottom; absolute intensities; ** contaminant originating from the α-KG preparation). ( b ) Gradient-selected heteronuclear multiple bond coherence spectra of the same U87IDHmut lysates acquired at 14 Tesla, confirming the production of [1- 13 C] 2-HG from [1- 13 C] α-KG. The 1 H– 13 C cross peaks of [1- 13 C] 2-HG (dotted box), confirm the [1- 13 C] 2-HG assignment at 183.9 p.p.m. Note: [1- 13 C] glycine was used as an external reference. ( c ) Temporal evolution of [1- 13 C] 2-HG in U87IDHmut cell lysate normalized to [5- 13 C] α-KG peak intensity, showing build-up of hyperpolarized [1- 13 C] 2-HG. Full size image Studies in orthotopic tumours Next, it was necessary to confirm that enough hyperpolarized [1- 13 C] α-KG is delivered and metabolized to produce detectable amounts of [1- 13 C] 2-HG in vivo, where [1- 13 C] α-KG needs to be delivered to the brain, cross the blood–brain barrier (BBB), penetrate the tumour and permeate the cell membrane. To this end, orthotopic tumours were implanted in the right putamen of athymic rats [31] . When tumours reached 0.38±0.15 cm 3 , hyperpolarized [1- 13 C] α-KG ( V =2 ml, c =100 mM) was injected intravenously. In a first experiment, dynamic 13 C spectra were acquired every 3 s from an axial slab including the whole tumour (2 cm thickness, Fig. 4a ). Data were acquired from the beginning of the intravenous injection using a multi-band variable flip angle (VFA) excitation scheme optimized to monitor 2-HG production by preserving the α-KG hyperpolarization and efficiently using the available magnetization to enhance the detection of 2-HG [34] , [35] . Hyperpolarized [1- 13 C] α-KG, hyperpolarized [1- 13 C] α-KG hydrate and a resonance at 184 p.p.m. were detected ( Fig. 4b ). The amount of [1- 13 C] α-KG in the slab was not significantly different between U87IDHwt and U87IDHmut animals, suggesting comparable delivery of the hyperpolarized substrate to the brain ( Fig. 4c ). Given the ≈1-p.p.m. linewidth of the 184-p.p.m. resonance in vivo , and in light of our findings in cell extracts showing that [5- 13 C] α-KG and [1- 13 C] 2-HG are only 0.1 p.p.m. apart, these two resonances could not be spectrally resolved. Nonetheless, we found a substantial difference in the temporal evolution of the 184 p.p.m. peak between mutant and wild-type IDH1 animals. In U87IDHwt animals, this resonance presents a unimodal temporal evolution centred around the time of maximum hyperpolarized [1- 13 C] α-KG (~10 s post injection) and probably corresponds to the hyperpolarized [5- 13 C] α-KG resonance originating from the injected solution ( Fig. 4d ). In contrast, the same resonance follows a bimodal temporal evolution in U87IDHmut animals, suggesting a delayed metabolic production of hyperpolarized [1- 13 C] 2-HG, with a maximum around 20 s ( Fig. 4d ). 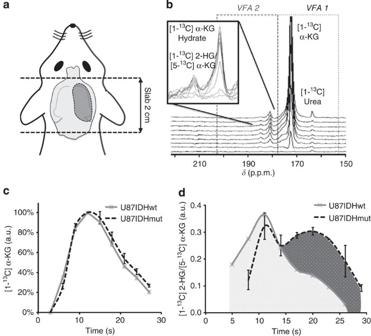Figure 4: Hyperpolarized 2-HG can be detectedin vivoin mutant IDH1 tumours. (a) Schematic of axial slab used forin vivodynamic13C MR experiments. The 2-cm slab was positioned to include the whole tumour while minimizing contamination from neck and nose blood vessels. (b) Stack plot ofin vivodynamic13C MR spectra acquired from a 2-cm slab following injection of hyperpolarized [1-13C] α-KG in a tumour-bearing U87IDHmut rat (temporal resolution 5 s; lb=20 Hz). A VFA scheme (VFA1/VFA2, see Methods) was used to improve the signal of hyperpolarized [1-13C] 2-HG. Signals from hyperpolarized [1-13C] α-KG (δC1-αKG=172.6 p.p.m.), hyperpolarized [1-13C] α-KG hydrate (δαKG-H=180.9 p.p.m.) and the resonance of hyperpolarized [1-13C] 2-HG/[5-13C] α-KG (δ=184 p.p.m.) are visible. (c) Integral of hyperpolarized [1-13C] α-KG as a function of time after its intravenous injection as measured from slab dynamic13C spectra acquired in U87IDHmut (black,n=3) and U87IDHwt (grey,n=2) tumour-bearing animals (error bars:±s.d.). (d) Integral of the 184-p.p.m. resonance ([1-13C] 2-HG/[5-13C] α-KG) as measured from slab dynamic13C spectra acquired in U87IDHmut (black,n=3) and U87IDHwt (grey,n=2) tumour-bearing animals (error bars:±s.d.). The bimodal temporal evolution of the composite resonance in U87IDHmut suggests metabolic production of hyperpolarized [1-13C] 2-HG. Figure 4: Hyperpolarized 2-HG can be detected in vivo in mutant IDH1 tumours. ( a ) Schematic of axial slab used for in vivo dynamic 13 C MR experiments. The 2-cm slab was positioned to include the whole tumour while minimizing contamination from neck and nose blood vessels. ( b ) Stack plot of in vivo dynamic 13 C MR spectra acquired from a 2-cm slab following injection of hyperpolarized [1- 13 C] α-KG in a tumour-bearing U87IDHmut rat (temporal resolution 5 s; lb=20 Hz). A VFA scheme (VFA1/VFA2, see Methods) was used to improve the signal of hyperpolarized [1- 13 C] 2-HG. Signals from hyperpolarized [1- 13 C] α-KG ( δ C1-αKG =172.6 p.p.m. ), hyperpolarized [1- 13 C] α-KG hydrate ( δ αKG-H =180.9 p.p.m.) and the resonance of hyperpolarized [1- 13 C] 2-HG/[5- 13 C] α-KG ( δ =184 p.p.m.) are visible. ( c ) Integral of hyperpolarized [1- 13 C] α-KG as a function of time after its intravenous injection as measured from slab dynamic 13 C spectra acquired in U87IDHmut (black, n =3) and U87IDHwt (grey, n =2) tumour-bearing animals (error bars:±s.d.). ( d ) Integral of the 184-p.p.m. resonance ([1- 13 C] 2-HG/[5- 13 C] α-KG) as measured from slab dynamic 13 C spectra acquired in U87IDHmut (black, n =3) and U87IDHwt (grey, n =2) tumour-bearing animals (error bars:±s.d.). The bimodal temporal evolution of the composite resonance in U87IDHmut suggests metabolic production of hyperpolarized [1- 13 C] 2-HG. Full size image We then examined the spatial distribution of hyperpolarized metabolites using a dedicated 2D 13 C chemical shift imaging (CSI) sequence [34] , [36] , [37] . Data were acquired from the beginning of the intravenous injection every 5 s with an in-plane spatial resolution of 5 mm. A multi-band excitation scheme was used to increase the signal of 2-HG by preserving the magnetization of its precursor α-KG [34] . The grid used for 2D CSI acquisition is shown as an overlay to a T2-weighted MR image for a U87IDHmut animal ( Fig. 5a ). Tumour volumes were not significantly different between U87IDHmut and U87IDHwt tumour-bearing animals (V wt =0.38±0.19 cm 3 versus V mut =0.38±0.12 cm 3 , unpaired Student’s t -test: P= 0.7). The levels of hyperpolarized [1- 13 C] α-KG were measured in tumour voxels (red/blue, n =6, including n =3 U87IDHmut and n =3 U87IDHwt), in normal brain voxels (green, n =6) and in blood-containing voxels centred on the basal artery (orange, n =6) for each imaging time point ( Fig. 5b ). As expected, the levels of hyperpolarized [1- 13 C] α-KG were significantly higher in blood-containing voxels as compared with normal brain (unpaired Student’s t -test: **P< 0.005 at 10, 15, 20 and 25 s; *P< 0.05 at 30 s). In addition, significantly higher levels of hyperpolarized [1- 13 C] α-KG were observed in the tumour voxels as compared with normal brain (unpaired Student’s t -test: **P< 0.005 at 10, 15, 20 and 25 s; *P< 0.05 at 30 s) and no significant differences in hyperpolarized [1- 13 C] α-KG levels were observed between tumour and blood-containing voxels, suggesting higher delivery and retention of hyperpolarized [1- 13 C] α-KG in the tumour region. This effect is consistent with increased angiogenesis, elevated vascular permeability and BBB breakdown in the tumour [31] , and probably enhances our ability to detect α-KG metabolism within the tumour region. Importantly, hyperpolarized [1- 13 C] α-KG levels were not significantly different between U87IDHwt and U87IDHmut tumours at any of the time points monitored ( Fig. 5c ), indicating that substrate delivery to tumour is independent of tumour IDH1 status, and is thus not a confounding factor in the detection of hyperpolarized [1- 13 C] 2-HG. 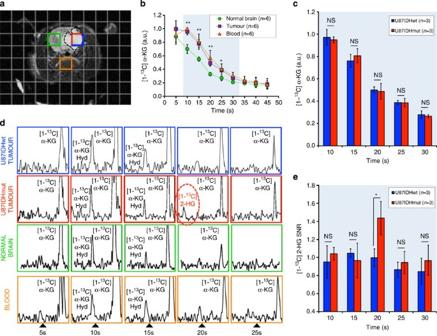Figure 5: Hyperpolarized α-KG is delivered and converted to 2-HGin situ. (a) T2-weighted anatomical MR image of U87IDHmut tumour-bearing animal overlaid with the grid used for 2D13C CSI acquisition (red/blue: tumour voxel; orange: blood voxel; green: normal brain voxel). (b) Time courses of hyperpolarized [1-13C] α-KG measured in tumour voxels (red/blue:n=6, includingn=3 U87IDHmut andn=3 U87IDHwt), in normal brain voxels (green:n=6) and in blood-containing voxels centred on the basal artery (orange:n=6; error bars:±s.d.). Significantly higher levels of hyperpolarized [1-13C] α-KG were observed in the tumour voxels as compared with normal brain (unpaired Student’st-test:**P<0.005 at 10, 15, 20 and 25 s;*P<0.05 at 30 s). (c) Levels of hyperpolarized [1-13C] α-KG measured in U87IDHwt (blue,n=3) and U87IDHmut (red,n=3) tumour voxels at 10, 15, 20, 25 and 30 s (error bars:±s.d.). No significant difference was observed at any time point. (d) Hyperpolarized13C MR spectra from one U87IDHwt tumour voxel (blue), one U87IDHmut tumour voxel (red), one normal brain voxel (green) and one blood voxel (orange) showing the temporal evolution of metabolites (no averaging performed; all spectra normalized to noise level). A resonance at 184 p.p.m. was observed at 20 s post injection of hyperpolarized [1-13C] α-KG only in the IDH1-mutant tumour voxel. (Note: the data presented from the U87IDHmut tumour, blood and normal brain voxels correspond to the U87IDHmut animal presented ina; the data from the U87IDHwt tumour are from an animal for which the MR image is not shown; Hyd, hydrate) (e) SNR of the 184-p.p.m. resonance measured in U87IDHwt (blue) and U87IDHmut (red) tumour voxels at 10, 15, 20, 25 and 30 s (error bars:±s.d.). A significant difference was found at 20 s post injection: SNR=1.4±0.2 in U87IDHmut tumours (n=3) versus SNR=1.1±0.1 in U87IDHwt tumours (n=3, unpaired Student’st-test:*P<0.05) consistent with this resonance corresponding to [1-13C] 2-HG. Figure 5: Hyperpolarized α-KG is delivered and converted to 2-HG in situ . ( a ) T2-weighted anatomical MR image of U87IDHmut tumour-bearing animal overlaid with the grid used for 2D 13 C CSI acquisition (red/blue: tumour voxel; orange: blood voxel; green: normal brain voxel). ( b ) Time courses of hyperpolarized [1- 13 C] α-KG measured in tumour voxels (red/blue: n =6, including n =3 U87IDHmut and n =3 U87IDHwt), in normal brain voxels (green: n =6) and in blood-containing voxels centred on the basal artery (orange: n =6; error bars:±s.d.). Significantly higher levels of hyperpolarized [1- 13 C] α-KG were observed in the tumour voxels as compared with normal brain (unpaired Student’s t -test: **P< 0.005 at 10, 15, 20 and 25 s; *P< 0.05 at 30 s). ( c ) Levels of hyperpolarized [1- 13 C] α-KG measured in U87IDHwt (blue, n =3) and U87IDHmut (red, n =3) tumour voxels at 10, 15, 20, 25 and 30 s (error bars:±s.d.). No significant difference was observed at any time point. ( d ) Hyperpolarized 13 C MR spectra from one U87IDHwt tumour voxel (blue), one U87IDHmut tumour voxel (red), one normal brain voxel (green) and one blood voxel (orange) showing the temporal evolution of metabolites (no averaging performed; all spectra normalized to noise level). A resonance at 184 p.p.m. was observed at 20 s post injection of hyperpolarized [1- 13 C] α-KG only in the IDH1-mutant tumour voxel. (Note: the data presented from the U87IDHmut tumour, blood and normal brain voxels correspond to the U87IDHmut animal presented in a ; the data from the U87IDHwt tumour are from an animal for which the MR image is not shown; Hyd, hydrate) ( e ) SNR of the 184-p.p.m. resonance measured in U87IDHwt (blue) and U87IDHmut (red) tumour voxels at 10, 15, 20, 25 and 30 s (error bars:±s.d.). A significant difference was found at 20 s post injection: SNR=1.4±0.2 in U87IDHmut tumours ( n =3) versus SNR=1.1±0.1 in U87IDHwt tumours ( n =3, unpaired Student’s t -test: *P< 0.05) consistent with this resonance corresponding to [1- 13 C] 2-HG. Full size image Hyperpolarized 13 C MR spectra from one U87IDHwt tumour (blue), one U87IDHmut tumour (red), one normal brain (green) and one blood voxel (orange) show the temporal evolution of hyperpolarized metabolites ( Fig. 5d ). The 184-p.p.m. resonance was observed only in the mutant IDH1 tumour voxel and appeared only at 20 s post injection ( Fig. 5d ). It was not observed in wild-type tumour or blood voxels, in spite of the comparable delivery of hyperpolarized [1- 13 C] α-KG in these three voxel types. On the basis of this data, we attributed the 184-p.p.m. resonance observed at 20 s in mutant IDH1 tumours to hyperpolarized [1- 13 C] 2-HG. When considering all the rats studied ( n =6), the SNR of hyperpolarized [1- 13 C] 2-HG was SNR [ 1 − 13 C] 2-HG mutt =1.4±0.2 in U87IDHmut tumours, whereas the resonance of hyperpolarized [1- 13 C] 2-HG was not detectable in any of the U87IDHwt tumours at that time point ( SNR [ 1 − 13 C] 2-HG wt =1.0±0.1; unpaired Student’s t -test: * P <0.05, Fig. 5e ). Consequently, although the SNR of hyperpolarized [1- 13 C] 2-HG was low, our results demonstrate statistical significance in discriminating between mutant IDH1 and wild-type tumours. These data also served to determine the in vivo effective decays of [1- 13 C] α-KG in U87IDHwt animals, in which no metabolism of α-KG to 2-HG was expected. The measured decays were 17.7±1.8 s in the vasculature and 20.6±1.7 s in the normal brain. As expected, these in vivo values are shorter than the in vitro measurements, as these decays include losses of polarization because of T 1 , flow and potentially metabolism [38] . U87IDHwt and U87IDHmut tumours of comparable size are shown in Fig. 6a . Heatmaps illustrate high levels of hyperpolarized [1- 13 C] α-KG in the blood vessels underneath the brain and in the tumours, regardless of tumour IDH1 status ( Fig. 6b ). In contrast, heatmaps of hyperpolarized [1- 13 C] 2-HG show the presence of 2-HG in U87IDHmut tumour only; this resonance is absent from blood-rich areas underneath the brain, from normal brain voxels and from U87IDHwt tumours ( Fig. 6c ). Similar findings were made in all U87IDHmut ( n =3) and U87IDHwt tumours ( n =3). 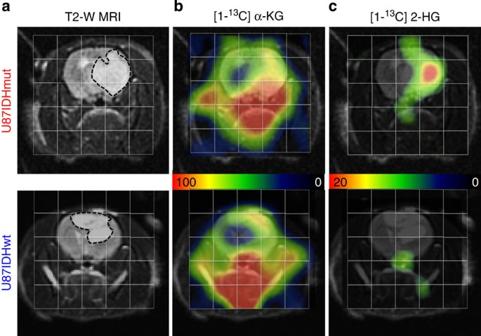Figure 6: Hyperpolarized 2-HG is detected only in mutant IDH1 tumours. (a) T2-weighted anatomical MR image of the head of a U87IDHmut (top) and a U87IDHwt (bottom) tumour-bearing animal overlaid with the grid used for 2D13C CSI acquisition. The tumours appear as hyperintense regions. (b) Corresponding heatmaps of hyperpolarized [1-13C] α-KG at 20 s post injection. (c) Corresponding heatmaps of hyperpolarized [1-13C] 2-HG at 20 s post injection, illustrating the presence of this metabolite in IDH1-mutant tumours only. Figure 6: Hyperpolarized 2-HG is detected only in mutant IDH1 tumours. ( a ) T2-weighted anatomical MR image of the head of a U87IDHmut (top) and a U87IDHwt (bottom) tumour-bearing animal overlaid with the grid used for 2D 13 C CSI acquisition. The tumours appear as hyperintense regions. ( b ) Corresponding heatmaps of hyperpolarized [1- 13 C] α-KG at 20 s post injection. ( c ) Corresponding heatmaps of hyperpolarized [1- 13 C] 2-HG at 20 s post injection, illustrating the presence of this metabolite in IDH1-mutant tumours only. Full size image Post-mortem analysis Immunohistochemical staining confirmed the presence of the mutant IDH1 isoform in U87IDHmut tumours but not in U87IDHwt ( Fig. 7a ). In line with these results, 2-HG was detectable using 1 H MRS only in the extracts of U87IDHmut tumours. The average level of 2-HG was 9.8±1.6 μmol g −1 of tumour ( n =3) and consistent with the estimated 10.1±2.5 μmol g −1 in cell lysates ( Fig. 7b ). 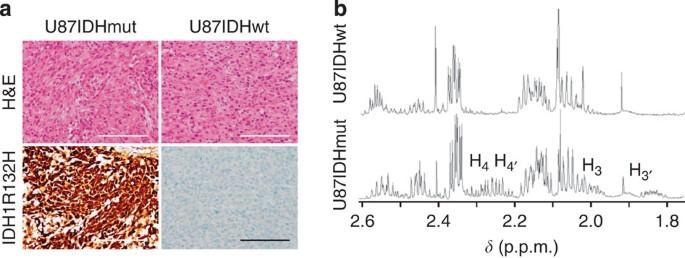Figure 7: Post-mortem analysis confirms the presence of mutant IDH1 and 2-HG. (a) U87IDHmut (left) and U87IDHwt (right) tumours had a similar histological appearance and were densely cellular on haematoxylin and eosin staining (H&E, top row). Immunostaining for mutant IDH1 (IDH1R132H, bottom row) demonstrated robust, diffuse positivity in U87IDHmut (left) tumours and no positive staining in U87IDHwt (right) tumours (magnification, × 200; scale bar, 100 μm). (b)1H MR spectrum of U87IDHwt (top) and U87IDHmut (bottom) tumour lysates acquired at 14 Tesla. The multiplets characteristic of 2-HG can be seen in the U87IDHmut spectrum not in the U87IDHwt (H3′=1.85 p.p.m.; H3=2.00 p.p.m.; H4,4′=2.25 p.p.m.; seeFig. 2for proton assignments). The level of 2-HG in U87IDHmut tumour extracts was 9.8±1.6 μmol g−1of tumour (n=3). Figure 7: Post-mortem analysis confirms the presence of mutant IDH1 and 2-HG. ( a ) U87IDHmut (left) and U87IDHwt (right) tumours had a similar histological appearance and were densely cellular on haematoxylin and eosin staining (H&E, top row). Immunostaining for mutant IDH1 (IDH1 R132H , bottom row) demonstrated robust, diffuse positivity in U87IDHmut (left) tumours and no positive staining in U87IDHwt (right) tumours (magnification, × 200; scale bar, 100 μm). ( b ) 1 H MR spectrum of U87IDHwt (top) and U87IDHmut (bottom) tumour lysates acquired at 14 Tesla. The multiplets characteristic of 2-HG can be seen in the U87IDHmut spectrum not in the U87IDHwt (H 3′ =1.85 p.p.m. ; H 3 =2.00 p.p.m. ; H 4,4′ =2.25 p.p.m. ; see Fig. 2 for proton assignments). The level of 2-HG in U87IDHmut tumour extracts was 9.8±1.6 μmol g −1 of tumour ( n =3). Full size image Our results show that hyperpolarized [1- 13 C] α-KG fulfills the mandatory requirements for a useful MR metabolic imaging probe. The T 1 relaxation time of [1- 13 C] α-KG in solution at 3 Tesla (52 s) compared favourably with the T 1 values of other commonly used DNP probes measured at 1.5–3 Tesla ([1- 13 C] pyruvate: T 1 ≈45–60 s [39] ; [1- 13 C] lactate: T 1 ≈45 s [40] ; and [1- 13 C] alanine: T 1 ≈40 s [41] ). The T 1 of such carbonyl-labelled DNP probes, including α-KG, is dominated by chemical shift anisotropy (CSA) relaxation processes. As a result, although lower magnetic fields lead to poorer spectral resolution, studies of hyperpolarized [1- 13 C] α-KG, like other hyperpolarized probes, benefit from lower field strengths at which the CSA is minimized (CSA-α B 0 2 ) and the T 1 is longer. The level of liquid state polarization (16% at 37 °C) was also comparable to the values reported for other hyperpolarized 13 C-carbonyl-labelled probes (range 7–30%) [27] . Achieving this polarization level required dissolving [1- 13 C] α-KG in a glassing agent (glycerol), at high concentration (5.9 M), and optimizing the concentrations of free radical and gadolinium agent. As our results show, the polarization level achieved using a Hypersense DNP system provided sufficient SNR for detection of hyperpolarized [1- 13 C] α-KG and its metabolic product, hyperpolarized [1- 13 C] 2-HG, in an animal in vivo . Further enhancements in polarization level could be achieved, thanks to newly developed equipment such as the GE SpinLab clinical polarizer, which has been shown to increase polarization levels by the use of a lower temperature and higher magnetic field for DNP [42] , [43] . A potential limitation of our study is the model system, which was genetically engineered to express mutant IDH1. We chose this approach because no models of clinical origin were available when we initiated our study. In fact, to date, only one tumour-forming model of clinical origin has been described [44] . Importantly, however, the levels of 2-HG detected in our tumour extracts (9.8±1.6 μmol g −1 of tumour) were comparable to the levels reported in patients (5–35 μmol of 2-HG per gram) [2] and studies of this model using 1 H MRS at high field strengths (7 and 14.1 Tesla) also detected 2-HG in vivo [22] , [23] . In light of these findings, we believe that the use of a genetically engineered model was justified for our proof-of-concept imaging study. Following in vitro injection of hyperpolarized [1- 13 C] α-KG into cell lysates, hyperpolarized [1- 13 C] 2-HG at 183.9 p.p.m. could be detected in U87IDHmut but not in U87IDHwt lysates. After intravenous injection, hyperpolarized [1- 13 C] α-KG was also detected in situ in orthotopic tumours, indicating that the probe was delivered to the brain and crossed the BBB in the tumour region. Some reports suggest that α-KG does not easily permeate the cell membrane [45] , whereas other studies show that brain cells are capable of taking up extracellular α-KG [46] . Our results demonstrate that, at least in our model, enough hyperpolarized [1- 13 C] α-KG permeates the tumour cells in vivo to enable the detection of its conversion to hyperpolarized [1- 13 C] 2-HG within a time frame compatible with a hyperpolarized 13 C MRS experiment. Further, our approach can serve to distinguish between mutant IDH1 and wild-type IDH1 tumours in vivo . Improvements in the delivery of hyperpolarized [1- 13 C] α-KG, as well as in the detection of hyperpolarized [1- 13 C] 2-HG, could be achieved by using alternative α-KG-based DNP probes. In particular, ester derivatives of α-KG, including octyl- and benzyl-esters have been reported to permeate the cell membrane more effectively [45] . Such derivatives would lead to increased intracellular α-KG concentrations and potentially higher levels of 2-HG, and might also enable studies of isocitrate dehydrogenase 2 within the mitochondria [46] , [47] . Previous studies indicate that the use of ester derivatives creates additional resonances than could hamper spectral differentiation [48] . However, preliminary studies in our lab investigating [1- 13 C] dimethyl-α-KG show that the compound resonates far from our spectral region of interest, and thus would not hamper 2-HG detection. Further, the natural abundance [5- 13 C] resonance of the ester was not detectable in our preliminary data, and, if present, would also be expected to resonate away from [1- 13 C] 2-HG. Our studies were enhanced by the use of innovative VFA and multi-band 13 C MR pulse sequences, which use the α-KG polarization efficiently while maximizing the signal of [1- 13 C] 2-HG and minimizing the signal from [5- 13 C] α-KG [34] , [35] , [36] , [37] . Specifically, [5- 13 C] α-KG originates from the injected hyperpolarized solution and is consequently present at early time points. In contrast, [1- 13 C] 2-HG is produced metabolically, and thus builds up at later time points. In our study, the multi-band sequence preserved the magnetization of [1- 13 C] α-KG by using a relatively low FA for its frequency but quenched the polarization of [5- 13 C] α-KG at the early time points by using a higher FA in that region. Further, the VFA scheme enhanced the signal of [1- 13 C] 2-HG at the later time points by increasing the FA over time. The use of such sequences is critical for enabling the direct detection of hyperpolarized [1- 13 C] 2-HG in vivo . When considering the possibility of future clinical translation, the dose of hyperpolarized α-KG needs to be considered. In the case of hyperpolarized pyruvate, the phase I clinical trial recently completed at UCSF [33] was based on a large number of animal studies in which 2 ml of 80 mM hyperpolarized pyruvate (~10 ml kg −1 , 0.8 mmoles of pyruvate per kg) was injected in rats [49] , and a comparable dose of 0.3 ml of 80 mM (~10 ml kg −1 , 0.8 mmoles of pyruvate per kg) was used in over 200 studies in mice, all with no adverse effects. In the clinical trial, the rodent studies were scaled in patients to a dose of 0.42 ml kg −1 of 250 mM pyruvate (0.1 mmoles of pyruvate per kg). Thus, volumes of 30–40 ml were injected, representing 1% of the total blood volume. These doses were very well tolerated with no dose-limiting toxicities and resulted in highly significant imaging results with a spatial resolution as low as 1 cm isotropic. In the case of α-KG, the concentration of hyperpolarized compound in our studies was limited by the technical requirements of the Hypersense hyperpolarizer (maximum volumes of substrate and dissolution buffer) resulting in a maximum achievable concentration of injected α-KG of 100 mM. However, the dose of α-KG used in this study (0.1 g kg −1 body weight) was 6.8 times lower (for a 200-g rat) than the no observed adverse effect level reported in rodents (NOAEL=1 g kg −1 body weight) [50] , and α-KG is sold in the United States as an over-the-counter nutritional supplement. Consistent with these facts, no adverse effects were observed in any of the animals included in our study ( n =11) and higher levels of α-KG could potentially be injected. However, as in the case of pyruvate, the concentration of α-KG would need to be increased to perform a similar study in patients with acceptable injection volumes. Recent studies demonstrate that total 2-HG levels can be monitored in vivo using 1D or 2D 1 H MRS in patients at clinical field strengths (1.5–3 Tesla) [18] , [19] , [20] , [21] . In an effort to compare 1 H MRS with our hyperpolarized 13 C approach for a potential clinical study, we performed an additional experiment, in which we compared the sensitivity of our rodent coil with the sensitivity of a 13 C human head coil array. The sensitivity of the human coil was lower by a factor of ~9. However, reported 1 H MRS studies were performed in voxel sizes of either 8 cm 3 , that is, ~16 times larger than our study (no SNR reported in post-processed data) [19] , [20] or 27 cm 3 , that is, ~54 times larger than our study (SNR=5) [18] . With such voxel sizes, we estimate that we would achieve an SNR of ~2.5 and ~8.4 on hyperpolarized [1- 13 C] 2-HG. Nonetheless, before clinical translation can be achieved, the approach presented in this proof-of-concept study will probably require further optimization to enhance [1- 13 C] 2-HG detection. Several areas of improvement can be envisaged. As mentioned above, the SpinLab clinical polarizer has been shown to enhance the achievable polarization levels [42] , [43] . This would increase the SNR of our hyperpolarized species, lead to better time-resolved kinetics and thus improve the detection of [1- 13 C] 2-HG. Higher concentrations of [1- 13 C] α-KG, or a more BBB and cell-permeable derivative of α-KG, could result in increased amounts of [1- 13 C] α-KG delivered to the tumour and, in turn, greater production of [1- 13 C] 2-HG (until the IDH1 enzyme is saturated). Finally, pulse sequences that would enhance the SNR of hyperpolarized [1- 13 C] 2-HG can be implemented. A non-dynamic 2D CSI sequence with a 90-degree FA at 20 s post injection would generate a higher SNR by a factor of ~3 compared with our current study, albeit at the detriment of temporal information. More promising is the recently developed 2D CSI sequence combining the multi-band and VFA scheme [35] , which would enhance the signal of [1- 13 C] 2-HG by using a progressively increasing FA. In addition, 1 H decoupling could be implemented to further increase the in vivo SNR of [1- 13 C] 2-HG, as previously reported [51] . Importantly, the information obtained by 13 C MRS is somewhat different from that obtained by 1 H MRS. 1 H MRS detects the total, steady-state, 2-HG levels present in both the extracellular and intracellular compartments [2] . In contrast, 13 C MRS dynamically informs on the metabolic fate of hyperpolarized [1- 13 C] α-KG. Accordingly, although we cannot rule out some residual enzymatic activity in necrotic regions [52] , 13 C MRS primarily probes the enzymatic activity of mutant IDH1 in live, metabolically active cells, and, as such, can inform in real-time on the presence of active mutant IDH1, 2-HG synthesis and its potential inhibition by novel therapies [14] , [15] . In summary, in this proof-of-concept study, we used 13 C MRS and were able to monitor the conversion of hyperpolarized [1- 13 C] α-KG into hyperpolarized [1- 13 C] 2-HG in cell lysates and, more importantly, in vivo in orthotopic brain tumours. Hyperpolarized [1- 13 C] α-KG presents a promising, non-radioactive and potentially clinically relevant agent for interrogation of IDH1 status in vivo . This innovative method provides information on IDH1 mutational status and activity in situ , it informs on real-time 2-HG production and complements the 1 H MRS methods that detect total steady-state 2-HG levels [18] , [19] , [20] . Additional optimization is required before clinical translation. Nonetheless, 13 C MRS of hyperpolarized [1- 13 C] α-KG could ultimately provide an additional valuable tool for diagnosis, prognosis, patient stratification, drug development and studies of response to emerging mutant IDH1-targeted therapies. Hyperpolarization of α-ketoglutarate [1- 13 C] α-ketoglutaric acid (2-oxoglutaric acid, Sigma-Aldrich, St Louis, MO) was dissolved in a mixture of water and glycerol (3:1 in volume), with 17.3 mM of OX63 trityl radical and 0.4 mM of Dotarem (Guerbet, France), to a final concentration of 5.9 M. A volume of 6.4 μl (cell lysate experiments) or 53 μl ( in vivo experiments) was polarized using a Hypersense polarizer (Oxford Instruments, Oxfordshire, UK) for ~1 h (3.35 Tesla, 1.4 K, 94.089 GHz). Following polarization, hyperpolarized [1- 13 C] α-KG was rapidly dissolved in a Tris-based isotonic buffer (pH=7.5±0.1) and used in this form for all experiments. Relaxation times and polarization levels A volume of 20 μl of [1- 13 C] α-KG was polarized as described above. Immediately after dissolution in an isotonic Tris-based buffer (40 mM Tris, 80 mM NaOH, 0.1 mg l −1 Na 2 EDTA) to obtain a 40-mM solution buffered at physiological pH, hyperpolarized [1- 13 C] α-KG was placed in a 5-ml syringe ( n =3, 3 Tesla Signa clinical MR system, GE Healthcare, Waukesha, WI) or in a 10-mm NMR tube ( n =3, 11.7 Tesla INOVA spectrometer, Agilent Technologies, Inc., Palo Alto, CA) and 13 C spectra were acquired using a 5-degree FA and a repetition time TR=3 s (parameters at 3 Tesla: number of transients (NT)=64, spectral width SW=5 kHz, 2,048 points; parameters at 11.7 Tesla: NT=300, SW=20 kHz, 4,000 points). For each field strength, the T 1 relaxation times of hyperpolarized [1- 13 C] α-KG ( δ C1-αKG =172.6 p.p.m. ), hyperpolarized [1- 13 C] α-KG hydrate ( δ αKG-H =180.9 p.p.m.) and hyperpolarized [5- 13 C] α-KG ( δ C5-αKG =184 p.p.m.) were determined by performing a monoexponential fit to the signal decay curve of the hyperpolarized compound [53] . Following complete decay of the hyperpolarized signal, a thermal spectrum with nearly identical parameters was acquired at 3 Tesla using a 90-degree FA and a repetition time of greater than 4 × T 1 (TR=10 s, NT=64; T 1 of solution shortened by adding 50 μl of Magnevist (Bayer Healthcare, Shawnee Mission, KS) to the hyperpolarized solution). The level of polarization in solution was calculated by comparing the first hyperpolarized spectrum with its corresponding thermal spectrum, correcting for FA and number of scans. The amplitude of the hyperpolarized signal was also corrected for T 1 relaxation during the transfer time from the polarizer to the spectrometer (~20 s). To evaluate the relaxation time T 1 of [1- 13 C] 2-HG, unlabelled L-2-hydroxyglutaric acid (Sigma-Aldrich) was dissolved in a mixture of water and glycerol (6:1 in volume), together with 17.3 mM of OX63 trityl radical and 0.4 mM of Dotarem (Guerbet). A volume of 100 μl was polarized using the Hypersense polarizer using the same conditions as for [1- 13 C] α-KG. After dissolution in 4 ml of Tris-based buffer (final pH=7.6), 13 C MR spectra of hyperpolarized 2-HG were recorded using the same parameters as the ones used for α-KG, except that the FA was 10° instead of 5°. Although the compound was not 13 C-enriched on the C1 position, the 1.1% natural abundance of 13 C was sufficient to generate a detectable hyperpolarized resonance at 183.9 p.p.m. The relaxation time T 1 of [1- 13 C] 2-HG at 3 and 11.7 Tesla was calculated as described above. Cell models Wild-type human IDH1 complementary DNA (MHS1010-58017, Open Biosystems, ThermoScientific) was mutagenized to generate an R132H-encoding cDNA using site-directed mutagenesis (Quick Change II, Applied Biosystems). Wild-type and mutant IDH1 cDNAs were then sub-cloned into separate green fluorescent protein-encoding lentiviral expression vectors. U87 GBM cells were obtained from the American Tissue Culture Collection and cells expressing exogenous wild-type or mutant IDH1 were created by introduction of lentiviral constructs encoding either the wild-type (U87IDHwt) or R132H IDH1 (U87IDHmut) cDNA, followed by selection of green fluorescent protein-positive cells by flow cytometry and verification for expression of the wild-type or mutant proteins by western blot using wild-type or R132H IDH-specific antibodies. Both modified U87 strains were cultured under standard conditions in high-glucose DMEM, (DMEM H-21, UCSF Cell Culture Facility, San Francisco, CA) supplemented with 10% heat-inactivated fetal bovine serum (Thermo Scientific Hyclone, Logan, UT), 2 mM L -Glutamine (Invitrogen, Carlsbad, CA), 100 U ml −1 penicillin and 100 mg ml −1 streptomycin (UCSF Cell Culture Facility). All cell lines in culture were maintained as exponentially growing monolayers at 37 °C in a humidified atmosphere of 95% air and 5% CO 2 . Western blotting Western blot analysis was performed on U87IDHmut and U87IDHwt cell lines to monitor IDH1 protein levels. Cytoplasmic proteins were electrophoresed on NuPAGE Novex 4-12% Bis-Tris gels (Life Technologies, Grand Island, NY) using the SDS–polyacrylamide gel electrophoresis method and electrotransferred onto polyvinylidene difluoride membranes. Blots were blocked and incubated with primary antibodies anti-IDH1wt (rabbit, number 3997, 1:1,000 dilution overnight; Cell Signaling Technology, Danvers MA) and anti-IDH1 R132H (mouse monoclonal H09 clone, 1:1,000 dilution overnight; Dianova, Miami, FL), and were then incubated with secondary antibody either anti-rabbit IgG (DyLight 800, 1:2,000; Cell Signaling Technology) or anti-mouse IgG (DyLight 680, 1:2,000; Cell Signaling Technology). The blots were visualized with a LI-COR Odyssey Infrared Imaging System (LI-COR Biosciences, Lincoln, NE). Spectrophotometric assay Mutant IDH1 activity was monitored in U87IDHmut and U87IDHwt cell lysates by adapting a spectrophotometric assay. For each cell type, ~2.0 × 10 7 cells were lysed in 400 μl of 50 mM Tris-based buffer with 1 μl ml −1 protease inhibitor cocktail (Sigma-Aldrich). Lysates were then homogenized by passing through a 27 gauge needle and sonicated on ice at 10% amplitude (3 × 5 s with 10 s intervals) using an FB505 20 kHz ultrasonicator (Fisher, Pittsburgh, PA). Cell lysates were centrifuged at 14,000 r.p.m. for 30 min at 4 °C. The supernatant was added to 1 ml of reaction buffer composed of 33 mM Tris-based buffer, 0.33 mM EDTA, 0.1 mM NADPH, 1.33 mM MnCl 2 and 1.3 mM α-KG (Sigma-Aldrich). A volume of 100 μl per well was then placed in a 96-well plate (Greiner Bio One, Monroe, NC). Absorbance at λ =340 nm was monitored every 10 s for 30 min using an Infinite m200 spectrophotometer (Tecan Systems, Inc., CA) and correlated to the concentration of NADPH [54] , [55] using a previously established calibration curve. For each lysate, the reaction rate R IDHmut of mutant IDH was calculated by linear regression of the first 300 s and reported in fmol of NADPH consumed per minute per cell ( n =3 per cell type). 1 H MRS of in cell lysates Approximately 1.5 × 10 8 U87IDHmut and U87IDHwt cells were extracted using the dual-phase extraction method [29] . 1D 1 H MRS spectra of U87IDHmut ( n =3) and U87IDHwt ( n =3) extracts were acquired on a 14-Tesla spectrometer (Bruker BioSpin Corporation, Billerica, MA) equipped with a 5-mm broadband probe. For 1D 1 H MRS, the following acquisition parameters were used: 90-degree FA, repetition time TR=2 s, SW=7194 Hz, 20,000 points, NT=100. All spectral assignments were based on literature reports ( http://www.hmdb.ca ) and confirmed by 2D 1 H MRS (2D total correlation spectroscopy sequence; f2: SW=20,000 Hz, 8,192 points; f1: SW=6,500 Hz, 64 points; mixing time 40 ms, WURST-8 adiabatic spin lock). 2-HG levels were quantified by peak deconvolution and integration using ACD/SpecManager 9 (Advanced Chemistry Development, Toronto, Ontario, Canada), correction for saturation and normalization to a trimethylsilyl propionate (TSP) reference and to cell number (Cambridge Isotope Laboratories, Andover, MA). Hyperpolarized 13 C MR studies of cell lysates A total of 1.2 × 10 8 U87IDHmut ( n =3) and U87IDHwt ( n =3) cells were extracted as described above. Lysates were placed in a 10-mm NMR tube and combined with a reaction buffer of similar composition to that used in the IDH1 spectrophotometric enzyme assay (while maintaining the same substrate concentrations per cell). In addition, MgCl 2 was used instead of MnCl 2 to prevent Mn 2+ -induced paramagnetic relaxation of nuclear hyperpolarization. Within 10 s of combining lysates and buffer, 1.2 ml of hyperpolarized [1- 13 C] α-KG dissolved in buffer (40 mM Tris, 9.4 mM NaOH, 0.1 mg l −1 Na 2 EDTA) was added to a final concentration of 4.7 mM. Immediately after injection, dynamic sets of hyperpolarized 13 C spectra were acquired on a 11.7-Tesla INOVA spectrometer (Agilent Technologies, Inc.) with a 13-degree FA for 300 s (TR=3 s, NT=100, SW=20 kHz, 40,000 points). After the total decay of the hyperpolarized signal, a 2D 1 H– 13 C gradient-selected heteronuclear multiple bond coherence spectrum of U87IDHmut cell lysate was recorded on a 14-Tesla Varian INOVA spectrometer (Agilent Technologies, Inc.) equipped with a 5-mm cryogenically cooled triple resonance inverse probe to confirm the [1- 13 C] 2-HG assignment: f2: SW=6903 Hz, 2,048 points; f1: SW=36,207 Hz, 4,000 points. 13 C pulse delays were 3.75 ms (to filter out one-bond coupling of 140 Hz) and 100 ms (optimal for 5 Hz 1 H– 13 C interactions). Tumour-bearing animals All animal research was approved by the Institutional Animal Care and Use Committee of the University of California, San Francisco. Athymic rats ( n =6 U87IDHmut, n =5 U87IDHwt, average weight 200 g, male, rnu/rnu homozygous, 5–6-week old at the time of intracranial injection; Harlan Laboratories, Indianapolis, IN) were used in this study. An hour before starting the intracranial injection, U87IDHwt or U87IDHmut cells were washed once with PBS solution, collected by trypsinization, counted and resuspended in serum-free McCoy’s medium to a final concentration of 3 × 10 5 cells per 10 μl. For intracranial injection, rats were anaesthetized by an intraperitoneal injection of a mixture of ketamine/xylazine (100/20 mg kg −1 , respectively). A volume of 10 μl of cell suspension was slowly injected into the right putamen of the animal brain by free-hand technique [56] . Buprenorphine (dose=0.03 mg kg −1 , V =600 μl) and bupivacaine (dose=5 mg kg −1 , V =300 μl) were injected subcutaneously right before injection of tumour cells for optimal pain management. In vivo -hyperpolarized 13 C MR studies In vivo experiments were performed on a 3-Tesla clinical MR system (GE Healthcare) equipped with a dual-tuned 1 H– 13 C transmit/receive volume coil (Ø I =40 mm). Rats were anaesthetized using isoflurane (1–2% in O 2 , 1.5 l min −1 ) and a 23 gauge catheter was secured in the tail vein for injection of hyperpolarized material. Anatomical imaging was performed to assess tumour location (2D fast spin echo, axial/coronal, TE/TR=20/1,200 ms, field of view=40 × 40 mm 2 , matrix 256 × 256, 20 slices, thickness=1 mm, acquisition time 5 min 7 s, NT=1). After 1 h, hyperpolarized [1- 13 C] α-KG was rapidly dissolved in isotonic buffer (40 mM Tris, 200 mM NaOH, 0.1 mg l −1 Na 2 EDTA) to obtain a 100-mM solution. Intravenous injection began within <20 s after dissolution. A volume of 2 ml of the hyperpolarized solution was injected over 12 s. Dynamic 13 C MR spectra were acquired from a 2-cm slab including the whole tumour on U87IDHwt ( n =2) and U87IDHmut ( n =3) tumour-bearing animals. The custom radiofrequency (RF) pulses were limited to this thickness by the demanding spectral and spatial selection requirements combined with gradient and RF hardware limitations of the clinical scanner. Nonetheless, this slice thickness provided full coverage for all tumours, which usually had an ellipsoid shape and grew preferentially along the anterior-posterior direction. The slab was positioned to minimize the contributions of neck and nose blood vessels. Data were acquired using an adiabatic double spin-echo sequence (TE/TR=35/3,000 ms) [36] . It used multi-band spectral-spatial RF excitation pulses with a VFA scheme that started with a smaller FA for [1- 13 C] α-KG (3.5°, VFA1) to preserve substrate magnetization and a larger FA for [1- 13 C] 2-HG/[5- 13 C] α-KG/[1- 13 C] α-KG hydrate (42.3°, VFA2) for improved SNR of 2-HG [34] . These FAs were progressively increased over time to efficiently use the hyperpolarized magnetization in the presence of metabolic conversion, with both VFA1 and VFA2 ramping up to a final 90-degree FA [35] . FA and frequency calibration was performed on a 0.6-ml syringe of 8 M [1- 13 C] urea placed next to the head. 13 C 2D dynamic CSI was acquired starting 5 s after the beginning of hyperpolarized [1- 13 C] α-KG injection in U87IDHwt ( n =3) and U87IDHmut ( n =3) animals using a sequence optimized for α-KG/2-HG [34] , [37] . This optimization included using a specialized multi-band spectral-spatial RF excitation pulse designed to provide a 4-degree FA for [1- 13 C] α-KG (to preserve substrate magnetization) and 25° elsewhere for improved SNR for 2-HG. An echo-planar spectroscopic imaging read-out gradient was used for increased imaging speed. This improves the SNR by reducing artifacts from T 1 decay, metabolic conversion and motion that can cause signal loss and blurring. The echo-planar spectroscopic imaging was optimized for maximum SNR efficiency while meeting the spectral bandwidth and spatial resolution requirements. Additional sequence parameters were adiabatic double spin-echo acquisition, bandwidth 543 Hz, resolution 10.4 Hz, 52 points, TE/TR=140/215 ms, matrix 8 × 18, 5 × 5 mm 2 resolution, slice thickness 2 cm, 1.7 s per image, images every 5 s. For all in vivo studies, B 0 shimming was performed using the automatic GE shimming routine, which acquires three orthogonal field maps and uses a least squares fit to set the linear shim gradients. The linewidth of [1- 13 C] α-KG was 26.3±9.8 Hz for the 1D MRS experiment (entire slab) and 23.0±3.4 Hz for the 2D CSI (brain voxel). 1 H decoupling was not applied; however, its use could increase the in vivo SNR of [1- 13 C] 2-HG in future studies, as illustrated by Marjanska et al. [51] In vivo MR data analysis Tumour volume was assessed from the anatomical T2-weighted images using the dedicated in-house SIVIC software ( http://www.sourceforge.net/projects/sivic/ ). For each animal, manual contouring of the tumour was performed for all axial slices and linear extrapolation was used to estimate final tumour volume. For in vivo slab dynamic experiments, integrals of hyperpolarized [1- 13 C] α-KG and [1- 13 C] 2-HG were quantified by peak integration of the dynamic hyperpolarized 13 C spectra using ACD/SpecManager 9 (Advanced Chemistry Development). The integrals were then corrected for the VFA schemes using Matlab (Mathworks, Natick, MA). For in vivo 2D CSI experiments, 13 C data sets were processed using SIVIC software to calculate the integrals of hyperpolarized [1- 13 C] α-KG and [1- 13 C] 2-HG and the s.d. of the noise to derive each metabolite SNR value. Superimposing the 2D 13 C CSI data onto the axial T2-weighted images was performed to localize the tumour voxels (estimated 68±27% of tumour tissue). Colour heatmaps of hyperpolarized [1- 13 C] α-KG and [1- 13 C] 2-HG were generated at 20 s after the start of injection by sinc-based spatial interpolation of the 2D 13 C CSI data to the anatomical image resolution using SIVIC. Post-mortem analysis of tumours One hour after the end of the last hyperpolarized 13 C MR experiment, animals ( n =5 U87IDHmut, n =4 U87IDHwt) were euthanized. Brains were resected and sectioned in the coronal plane to bisect the tumour. The posterior sections of the brains were placed in 10% buffered formalin for 24 h, and then moved to 70% cold ethanol. The sections were then embedded in paraffin and sectioned in the axial plane. Sections were stained with haematoxylin and eosin and immunostained for mutant IDH1 (IDH1 R132H ) using a mouse monoclonal anti-IDH1 R132H (DIA H09; Dianova) at 1:50 dilution. All stained slides were imaged using an Olympus BX41 microscope and Olympus DP72 camera and assessed qualitatively. The anterior sections of the brains were dissected to isolate the tumour from the normal brain tissue, and tumours were quickly snap-frozen in liquid N 2 . Tumour tissues were then extracted using the dual-phase extraction method [57] . After lyophilization, tumour extracts were reconstituted in 400 μl D 2 O in a 5-mm NMR tube and 1D 1 H MR spectra were recorded on a on a 14-Tesla Varian INOVA spectrometer (Agilent Technologies, Inc.) using the following parameters: 90-degree FA, TR=2 s, SW=7194 Hz, 20,000 points, NT=128. In vivo 2-HG levels were quantified by peak deconvolution and integration using ACD/SpecManager 9 (Advanced Chemistry Development), correction for saturation and normalization to a TSP reference and to grams of tumour tissue (Cambridge Isotope Laboratories). Coil sensitivity in rodents versus humans In an effort to estimate the achievable SNR of hyperpolarized [1- 13 C] 2-HG in a patient brain tumour, we needed to account for the decreased sensitivity of the larger coils required for patient studies. To this end, we compared the sensitivity of the rodent coil used in our study with the sensitivity of a human 13 C head coil array used for clinical brain imaging (eight-channel custom coil array with two 18 cm linear panels; four surface coils per panel; rectangular coil element 5 × 10 cm) [58] . A 0.6-ml sealed syringe containing 8 M [1- 13 C] urea was positioned in the center of each of the two coils and an identical pulse-acquire sequence was applied to measure the [1- 13 C] urea signal (90-degree FA, NT=64). The decrease in sensitivity in the human coil was assessed by direct comparison of the amplitudes of the [1- 13 C] urea signal in human versus rodent coil. Statistical analysis All results are expressed as mean±s.d. The unpaired two-tailed Student’s t -test was used to determine statistical significance of the results, with a P -value<0.05 considered as significant. How to cite this article: Chaumeil, M. M. et al. Non-invasive in vivo assessment of IDH1 mutational status in glioma. Nat. Commun. 4:2429 doi: 10.1038/ncomms3429 (2013).